The role of MHC supertypes in promoting trans-species polymorphism remains an open question Phylogenetic analysis The relationships between 539 MHC class II exon 2 alleles reported in the Supplementary Data 1 of Lighten et al. [1] were reconstructed from full 209 bp nucleotide sequences using the neighbor Joining method in MEGA 7 [11] . The matrix of evolutionary distances was computed using the Jukes–Cantor method. The robustness of the relationships was assessed with 500 bootstrap replicates. Population genetics We downloaded Lighten et al.’s population-genetic data and analysis scripts from Ben J. Ward’s GitHub repository for the paper ( https://github.com/BenJWard/Supertypes_RedQueen_TSE ) on 17/04/2017, and followed their annotated analysis to produce the data used for Supplementary Fig. 2 and the top-left panel of Supplementary Fig. 1 . This analysis first calculates the observed MHC D EST [12] between all population pairs in the dataset, and uses each population’s mean pairwise D EST as the red, ‘observed’ dots in the plots. This is followed up by reassigning alleles to supertypes at random, keeping the number of alleles in each supertype constant, and then recalculating each population’s mean pairwise D EST . The means of 1000 repeats of this randomisation become the blue, ‘expected’ dots in the respective figures, with the standard deviations used for the blue dots’ error bars. Conceptually, the blue dots and their error bars represent a scenario in which there is no selection at the supertype level, i.e. supertype population genetics are a reduced-diversity reflection of allele-based population genetics. An observed supertype-based population structure stronger than this neutral expectation would imply diverging selection on supertypes, whereas lower population structure would imply balancing/stabilising selection. We then repeated these analyses removing each supertype in turn, i.e. removing all instances of all alleles in the focal supertype, and thereby any individuals that were homozygous for the focal supertype. One population (Cumana, n = 6) was homozygous for ST13 and was removed from that supertype’s analysis. 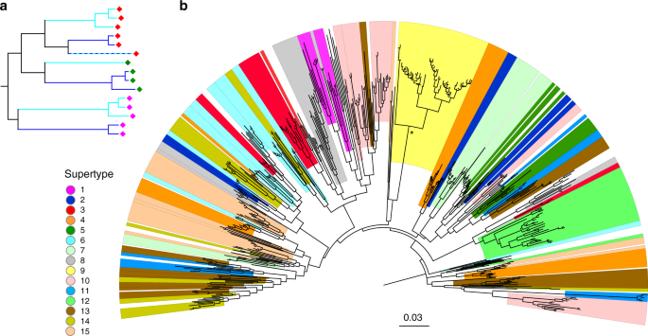Fig. 1 Predictions and results of phylogenetic analysis.aThe hypothetical pattern expected if balancing selection on supertypes maintains TSP, but alleles within supertypes experience rapid turnover. Hypothetical supertypes are marked with diamonds of the same colour, and the species-specific branches are in turquoise and deep blue. Supertype lineages should be shared between species, but sharing of identical alleles (dashed line) should be rare.bNeighbour-joining tree of 539 MHC class II exon 2 alleles reported by Lighten et al.1. The tree was constructed from a matrix of Jukes–Cantor distances calculated using all 209 nucleotide positions. Alleles from each supertype are marked with the same colour as in Lighten at al. Supertype 9 is marked yellow; the asterisk indicates that it is the only monophyletic supertype (bootstrap support 97%) 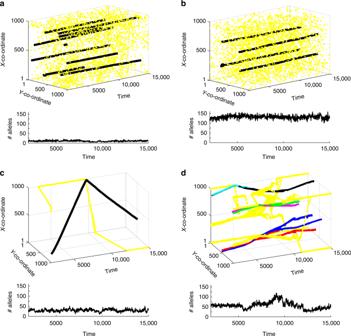Fig. 2 Results of simulations based on the model proposed by Lighten et al. Parasite haplotypes (yellow) and host supertypes (black and other colours) are represented as coordinates in 1000 × 1000 grid, reflecting their functional properties (the closer a parasite is to the host, the more likely is a successful host immune response). Each panel shows how changes in specified parameters in the model, compared to the parameters used by Lighten et al. to produce their Fig. 4, affect the outcome (parameters other than stated in the description are as in Lighten et al.).aMutation rate set to 10−2for pathogens and 10−3for hosts, population size increased to 100,000. In contrast to the results reported by Lighten et al. using much higher mutation rates, the effective number of alleles maintained in a population is small.bSelection on parasites (but not on hosts) ‘turned off’. This simulation gives the most similar outcome to that reported by Lighten et al., despite the lack of host-parasite coevolution (see Supplementary Fig.6for the scenario with no random pathogen genotypes added).cSimulations that do not seed each pathogen generation with ≈100 new genotypes, but mutation parameters as in Lighten et al. Host-parasite coevolution utilizing mutational variance alone does not maintain several stable supertypes, even though the simulations started from creating a set of random MHC alleles and pathogens in the same way as Lighten et al.dParameters as inc, but 10 independent parasites simulated. Several supertypes are observed at any time point, but they are not stable through time. Effective number of alleles (#alleles) has been calculated for a sample of 100 individuals to allow comparison with the results of Lighten et al. The simulations were written in MatLab and the algorithm follows that described by Lighten et al. The MatLab code is provided in our Supplementary Data1 To compare the effects of removing each supertype, we calculated the mean and SD of the difference between the red and blue dots for each jack-knifed dataset (second column of Supplementary Table 1 ). We also calculated the Spearman correlation coefficient between each jack-knifed dataset’s red dots and the red dots of the full dataset (third column of Supplementary Table 1 ). To assess the degree to which each supertype’s jack-knifed dataset might be influenced by supertype membership size (number of alleles) or supertype frequency, we performed three additional sets of randomised deletions for each supertype. In the first, we repeatedly removed all occurrences of a random subset of unique nucleotide sequences from the dataset, corresponding in size to the number of sequences in the focal supertype (columns 7–8 of Supplementary Table 1 ). In the second, we made randomized deletions that matched the frequency of the focal supertype but without systematically removing any particular nucleotide sequences (columns 9–10 of Supplementary Table 1 ). The third was a spatially structured version of the second, matching the number of random deletions within each population to the frequency of the focal supertype within each population (columns 11–12 of Supplementary Table 1 ). Simulations To analyze the theoretical results of Lighten et al. we first reconstructed the simulation model of immune gene evolution presented in their work [1] ; the detailed description of the model can be found in the Lighten et al. We then tested their model in an extended parameter space of pathogen mutation rate, host mutation rate and population size, as specified in our figures. Additionally, we ran simulations in three scenarios not considered by Lighten et al. In the first, we removed the feature of Lighten et al. 's simulations that seeded pathogen population with 1% of random genotypes (‘random’ meaning randomly distributed in physicochemical parameter space) every host generation. The second was a neutral scenario in which parasites were sampled randomly every generation, i.e. without taking into account their ability to infect hosts, thereby preventing parasite adaptation. The third extended simulations of Lighten et al. by including more than one pathogen co-evolving with one host species. The algorithm of the simulation model used in our work can be found in Supplementary Data 1 . Code availability The code for our simulations is available in Supplementary Data 1 .